Electrofluorochromism in π-conjugated ionic liquid crystals Materials in which photoluminescence is modulated by redox processes are known as electrofluorochromic. Intrinsically switchable fluorophores, incorporating both redox and fluorescent moieties, could be ideal electrofluorochromic materials if they possess high fluorescence quantum yields in at least one of their redox states. Fluorescent liquid crystals with redox active centres could combine the above requirements with the advantage to work in bulk anisotropic phases. However, electrofluorochromic liquid crystals have not been reported yet because their synthesis is challenging due to aggregation-caused fluorescent quenching. Here we show the first examples of electrofluorochromic π-conjugated ionic liquid crystals based on thienoviologens. These ordered materials, combining ionic and electronic functions, are highly fluorescence in the bulk state (quantum yield>60%). Their direct electrochemical reduction leads to fast and reversible bulk electrofluorochromic response in both columnar and smectic phases allowing for fluorescence intensity modulation and colour tuning. Materials able to switch their photoluminescence in response to various external stimuli can be potentially used for memory devices, sensors, security materials and informational displays [1] , [2] , [3] , [4] , [5] , [6] . Specifically, materials in which photoluminescence is modulated by redox processes are known as electrofluorochromic [7] . They can be broadly classified into switchable molecular dyads and intrinsically switchable electroactive fluorophores [8] . In the first case, the fluorophore is linked to a redox moiety that acts as fluorescence switching through energy [9] , [10] or electron transfer mechanisms [11] , [12] , [13] , [14] . In the latter, electrochemical fluorescence switching is enabled on direct reduction or oxidation of the fluorophore (either small molecules or conjugated polymers) [15] , [16] , [17] , [18] . Electrofluorochromism is usually coupled to electrochromism of the redox unit in dyads or of the electroactive fluorophore. The more straightforward way to electrofluorochromism is the direct electrochemical fluorescence switching through the formation of ion and neutral radicals. However, while the latter are not fluorescent or exhibit very low fluorescence, the first ones are usually not stable and their electrochemically monitoring is challenging [8] . Such main limitations have hampered the development of this class of molecules. Fluorescent liquid crystals with redox active centres could combine the above requirements with the advantage to work in bulk anisotropic phases. However, the synthesis of fluorescent liquid crystal including ionic ones, is challenging because of aggregation-caused fluorescent quenching [19] , [20] , [21] , [22] . Thus, electrofluorochromic liquid crystals have not been reported yet. Here we propose a novel approach with thienoviologens 4,4′-(2,2′-bithiophene-5,5′-diyl)bis(1-alkylpyridinium)triflimide compounds 1 and 2 with flexible, promesogenic alkyl chains of 9 and 11 carbon atoms, respectively ( Fig. 1a ). Their design has been specifically conceived to combine the electrochromic and fluorescent properties of thienoviologens in solution [23] , [24] , with the supramolecular organization arising from their liquid crystalline properties. Indeed, these compounds exhibit a unique bismesomorphism, self-assembling into either columnar or calamitic phases, depending on the alkyl chains’ length and on the temperature ( Fig. 1a ) [25] . We report the optical, electrochemical and spectroelectrochemical properties of these LC materials in the bulk phase. Notably, they exhibit high fluorescence quantum yields (up to 68%) amongst the highest ever reported, either at room temperature or in the mesophase. Moreover, they are strong electron acceptors showing two reduction processes at −0.68 and −1.17 V versus Ag + /Ag. Their electrochemical reduction is achieved by an efficient electron hopping mechanism through the π-conjugated system of the LC state coupled to a high ionic conductivity (10 −4 S cm −1 ) through ion channels formed within the nanosegregated LC phases. On the application of reductive voltages, the materials show fast and reversible electrochromic and electrofluorochromic responses. They allow for full control on the modulation of the fluorescent intensity with fluorescence contrasts (ΔFL) of up to 80% and short switching times (<3.5 s). Here we report also that the application of an electric field on the isotropic liquid state of compound 2 induces the transition into the smectic phase that is observed under polarized optical microscope (POM) and is reflected in a hard red shift of the fluorescence spectrum of the material. This completely reversible phenomenon allows for colour tuning of the fluorescence. 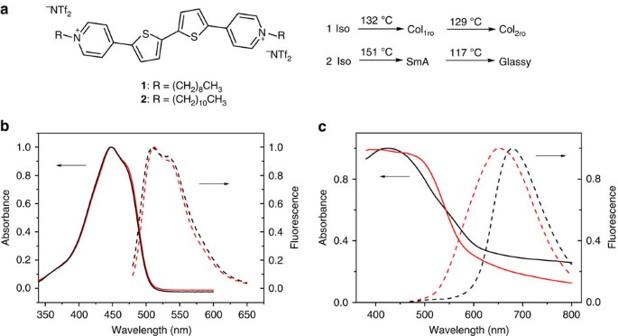Figure 1: Thienoviologens investigated and their photophysical properties. (a) Molecular structures and mesophase behaviour on cooling from the isotropic liquid state (Iso=isotropic liquid state; Colro=rectangular ordered columnar phase; SmA=Smectic A phase)25. (b) Optical absorption and fluorescence spectra of1(solid line) and2(dot line) in dichloromethane (DCM) solution. (c) Optical absorption and fluorescence spectra of 1 (red lines) and 2 (black lines) in 7 μm thick films at room temperature. Figure 1: Thienoviologens investigated and their photophysical properties. ( a ) Molecular structures and mesophase behaviour on cooling from the isotropic liquid state (Iso=isotropic liquid state; Col ro =rectangular ordered columnar phase; SmA=Smectic A phase) [25] . ( b ) Optical absorption and fluorescence spectra of 1 (solid line) and 2 (dot line) in dichloromethane (DCM) solution. ( c ) Optical absorption and fluorescence spectra of 1 (red lines) and 2 (black lines) in 7 μm thick films at room temperature. Full size image Bulk photophysical properties of LC thienoviologens Table 1 summarizes some photophysical properties of 1 and 2 . In solution they absorb at 430 nm and are highly fluorescent at 530 nm ( Table 1 ), irrespective of the length of the alkyl chains ( Fig. 1b ). Much more interesting, however, are their photophysical properties in the bulk phase. The room temperature thin-film absorption and emission spectra of both materials show broader and slightly red-shifted (~40 nm) absorption bands and hardly red-shifted emission bands (>100 nm) with respect to those in solution ( Fig. 1c ). Table 1 Photophysical properties of compounds 1 and 2. 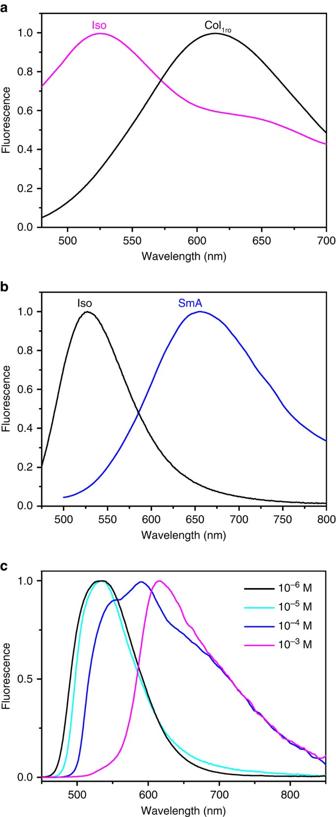Figure 2: Aggregation-caused fluorescence shift. Bulk emission spectra of a thin film of (a),1in the Iso state (magenta line) and in the Col1rophase (black line) and (b),2in the Iso state (black line) and in the SmA phase (blue line). (c) Concentration dependence of the fluorescence spectra of1in DCM solution. Full size table Figure 2a,b shows the bulk emission spectra of thin films of 1 and 2 on cooling from the isotropic liquid state. The melt shows an emission band at about 540 nm, which resembles that found in solution suggesting that this band is characteristic of the single molecule. However, the supramolecular organization introduced on cooling by entering the mesophase gives rise to a new emission band at about 670 nm and to the progressive disappearing of that at 530 nm (see also the spectrum at room temperature in Fig. 1c ). This very large red shift of the fluorescence emission (~140 nm) is caused by the aggregation of the molecules into the mesophase. An analogous ‘aggregation-caused shifting’ is also observed in solution by increasing the thienoviologen concentration, as shown in Fig. 2c . Indeed, the fluorescence emission band at 530 nm, typical of dilute solutions (<10 −5 M), systematically shifts to higher wavelengths with increasing concentration, until it disappears above 10 −4 M and a new band at about 600 nm occurs. These spectral changes indicate that molecular aggregates start to form in solution at an onset concentration of about 10 −4 M where the emission spectral features of both single molecules (530 nm) and aggregates (620 nm) are detected. For concentrations larger than 10 −4 M, the emission spectrum of the solution exhibits only a band at 620 nm; thus, it is essentially dominated by the fluorescence of the aggregated state ( Fig. 2c ). Figure 2: Aggregation-caused fluorescence shift. Bulk emission spectra of a thin film of ( a ), 1 in the Iso state (magenta line) and in the Col 1ro phase (black line) and ( b ), 2 in the Iso state (black line) and in the SmA phase (blue line). ( c ) Concentration dependence of the fluorescence spectra of 1 in DCM solution. Full size image It is worth highlighting that compounds 1 and 2 exhibit high fluorescent quantum yields (Φ) either in the liquid crystalline phases or in the solid state at room temperature ( Table 1 ), among the highest ever reported [19] , [20] , [21] , [22] . Bulk electrochemical properties The bulk optical properties of materials 1 and 2 are strongly affected by a direct current (dc) electric field. Actually, the dications of 1 and 2 are electron deficient and can be easily reduced to the neutral form either in solution, by a single two-electron reduction step ( Supplementary Fig. 2 ) [24] , or in the bulk. Their redox properties in the liquid crystalline phase were determined here in a three-electrode cell on thin films of the materials (40 μm) sandwiched between two indium-tin-oxide (ITO) glass electrodes. A thin Ag wire (16 μm), placed between the ITO electrodes, served as reference ( Fig. 3a ). 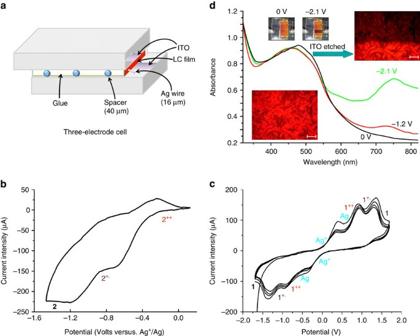Figure 3: Bulk electrochromism of LC thienoviologens. (a) Three-electrode liquid crystalline cell. (b) CV of2in the SmA phase (142 °C; scan rate 35 mV s−1; electrode area 0.20 cm2). (c) CVs of1in the columnar phase (120 °C; scan rate 35 mV s−1; electrode area 0.15 cm2). (d) Optical absorption spectra of2in the SmA phase at 0 V (black line), at −1.2 V (red line) and at −2.1 V (green line). Insets indshow POM images of the SmA phase at 0 V (lower image) and −2.1 V (upper image; scale bars=50 μm). Note that in the ITO-etched area (not conductive) of the LC cell the material is not dark coloured. Figure 3b shows a representative standard cyclic voltammogram for material 2 in the SmA phase. Under these conditions, two quasi-reversible one-electron reduction peaks at −0.68 and −1.17 V versus Ag + /Ag are observed. They are, respectively, attributed to the radical cation and the neutral species. Figure 3: Bulk electrochromism of LC thienoviologens. ( a ) Three-electrode liquid crystalline cell. ( b ) CV of 2 in the SmA phase (142 °C; scan rate 35 mV s −1 ; electrode area 0.20 cm 2 ). ( c ) CVs of 1 in the columnar phase (120 °C; scan rate 35 mV s −1 ; electrode area 0.15 cm 2 ). ( d ) Optical absorption spectra of 2 in the SmA phase at 0 V (black line), at −1.2 V (red line) and at −2.1 V (green line). Insets in d show POM images of the SmA phase at 0 V (lower image) and −2.1 V (upper image; scale bars=50 μm). Note that in the ITO-etched area (not conductive) of the LC cell the material is not dark coloured. Full size image It is noteworthy that film thicknesses smaller than those used in the three-electrode cell are desirable for a better mesophase assembling. This condition improves the electro-optical response of the material, avoiding also problems related to detector saturation in optical absorption spectroscopy. Therefore, a two-ITO-electrode cell with smaller cell gaps (~7 μm) was conveniently used for electrochromic and electrofluorochromic studies. The reduction potentials of materials 1 and 2 in the two-electrode cell ( Fig. 3c ) are shifted of about −0.4 V with respect to their standard values referenced to Ag + /Ag ( Fig. 3b ). This can be seen by comparing the standard cyclic voltammogram ( Fig. 3b ) with that reported in Fig. 3c , acquired with a two-electrode cell. In this case, the Ag film was used as internal standard for a proper comparison. Three reduction processes can be seen at ±0.36, ±0.94 and±1.33 V, respectively, related to the reduction of Ag + , 1 ++ and 1 +. ions. Therefore, in the symmetric two-electrode cell, material reduction alternately occurs at both ITO electrodes and the original dication species is completely recovered after each return sweep cycle ( Fig. 3c ). The inversion of the sign of the potential changes the ITO electrode from which electrons are injected into the material. Bulk electrochromism The formation of the reduced species gives rise to new absorption bands in the visible region from 550 to 800 nm involving a colour change of the materials (both columnar and smectic) from red to almost black ( Fig. 3d ). Reduction of the thienoviologen cations in the liquid crystalline phase does not alter the texture of the mesophase. This can be clearly seen under a polarized optical microscopy during the application of the reducing dc voltage. An example is shown in the inset of Fig. 3d and Supplementary Movie 1 where it can be seen that the smectic layers are preserved in the dark cell region where reduction took place. This phenomenon is completely reversible and the original colour is restored when a 0-V is biased. Here an electrochromic response in the bulk LC phases is observed in electron acceptor π-conjugated ionic liquid crystals (ILCs), while a similar behaviour has been reported only by Kato and colleagues for hole-conducting ILCs self-segregating in SmA phases [26] , [27] . As previously suggested by Kato and colleagues, electrochromism in π-conjugated ILCs is possible because of the coupling of electronic and ionic functions in the nanosegregated structure of ILCs [26] , [27] . Electron injection at the cathode causes the reduction of the thienoviologen dication and the reduced species is transferred to the anode by electron hopping via π–π intermolecular interaction through the film. At the same time, electrode depolarization occurs due to the transportation of the bistrifliimide anions towards the anode. This mechanism implies a relatively high ionic conductivity of the liquid crystalline materials without the need for an external electrolyte. We have preliminary measured ionic conductivities of compounds 1 and 2 perpendicular to the long molecular axis (planar alignment conditions), by electrochemical impedance spectroscopy using the ITO liquid crystalline cell as a parallel plate capacitor ( Supplementary Fig. 3 ) [28] , [29] . Conductivity values as high as 10 −4 S cm −1 were found, indicating that mesophase nanosegregation effectively create ion conducting pathways within the materials. Bulk electrofluorochromism The coupling of fluorescent and electrochromic properties in these LC thienoviologens leads to unique electrofluorochromic-ordered materials. Indeed, when dc reductive voltages are biased between the ITO electrodes of the LC cell, direct electrochemical switching of the fluorescent intensity (~10-fold increase) occurs in both mesophases ( Fig. 4a,b ). The electrofluorochromism in these systems induces also a slight shift of the emission wavelength ( Fig. 4 a,b ). Notably, this effect is highly increased in the isotropic phase of 2 , allowing for colour tuning from green to red. Indeed, as shown in Fig. 5a , when a reductive voltage is applied on 2 in the isotropic liquid state (Iso), the characteristic emission band at 540 nm disappears and a strong band at about 610 nm takes place. This profound change of the fluorescence spectrum from that typical of the melt material into that typical of the structured phase is similar to the aggregation-caused shifting effect shown in Fig. 2a,b and suggests a field-induced molecular ordering. Indeed, monitoring it under POM on the application of the electric field, we observe the instantaneous formation of bâtonnets and, after a few seconds, the fan-shaped texture of the smectic A phase ( Fig. 5b–f and Supplementary Movie 2 ). On the other hand, the huge intensity of the band at 610 nm compared with that of the Iso state ( Fig. 5a ), should be attributed to the electrochemical switching of the fluorescent intensity ( Fig. 4a,b ). 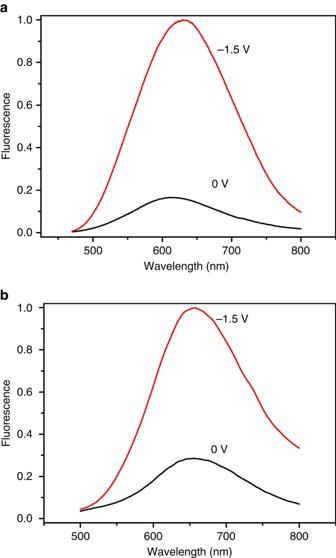Figure 4: Bulk electrofluorochromism. (a) Fluorescence spectra at 0 V (black line) and −1.5 V (red line) of thin films (10 μm thick) of1in the columnar phase and (b)2in the smectic phase. Figure 4: Bulk electrofluorochromism. ( a ) Fluorescence spectra at 0 V (black line) and −1.5 V (red line) of thin films (10 μm thick) of 1 in the columnar phase and ( b ) 2 in the smectic phase. 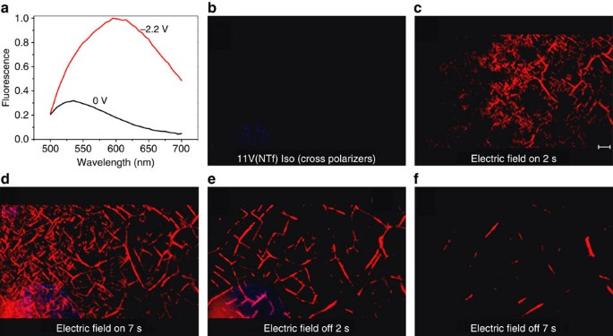Figure 5: Fluorescence colour tuning by electric field-induced transition effect. (a) Fluorescence spectrum of a thin film of2(15 μm thick) in the isotropic liquid state (black line). On the application of a −2.2-V potential, the spectrum is hardly red-shifted (red line) due to the electric field-induced transition from the Iso state to the SmA phase. (b–f) Temporal sequence of POM images acquired at 170 °C illustrating the electric field (1,500 V cm−1) -induced Iso/smectic phase transition (scale bar=40 μm; see alsoSupplementary Movie 2). Full size image Figure 5: Fluorescence colour tuning by electric field-induced transition effect. ( a ) Fluorescence spectrum of a thin film of 2 (15 μm thick) in the isotropic liquid state (black line). On the application of a −2.2-V potential, the spectrum is hardly red-shifted (red line) due to the electric field-induced transition from the Iso state to the SmA phase. ( b – f ) Temporal sequence of POM images acquired at 170 °C illustrating the electric field (1,500 V cm −1 ) -induced Iso/smectic phase transition (scale bar=40 μm; see also Supplementary Movie 2 ). Full size image Interestingly, the Iso/mesophase field-induced transition process is not observed for compound 1 (Iso/columnar), suggesting that it is strongly dependent on the nanosegregation of the LC structures. Therefore, this phenomenon deserves further investigation for its full comprehension. Electrofluorescence switching The electrofluorochromic response was monitored at 630 nm as a function of time during the application of a voltage potential step. It is useful to recall that these measurements were performed in a front-face geometry (see Methods section) and that electrons were injected onto the ITO surface illuminated by the excitation source to detect the fluorescence response of the first electroreduced material layers. It can be seen that the fluorescence emission starts rapidly to increase from the baseline value when the potential step is switched on and grows up to 10 times the baseline until the potential is switched off (after 10 s). Then, it decays back to the baseline when the potential is set to 0 V ( Fig. 6a ). It is further noted that this increase cannot be due to an increase of the absorbance of the reduced species with respect to that of the dication at the excitation wavelength (450 nm), as clearly shown in the absorption spectra reported in Fig. 3d . 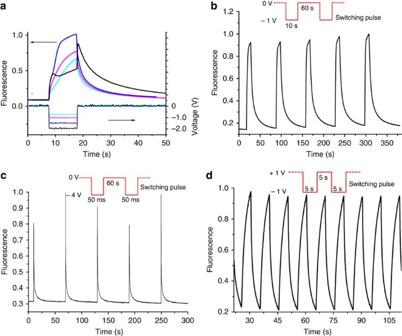Figure 6: Reversible fluorescent switching monitored at 630 nm. (a) Fluorescence switching of1in the Col1rophase on the application of −0.7 V (turquoise line), −1.0 V( magenta line), −1.5 V (blue line) and −2.0 V (black line) for 10 s. (b) Repetitive switching cycles of1in the Col1rophase between −1.0 V for 10 s and 0 V for 60 s (delay time between pulses) and (c) −4.0 V for 50 ms and 0 V for 60 s delay time between pulses. (d) Fluorescence switching of2in the SmA phase between −1.0 and +1.0 V for a step duration of 5 s. Figure 6: Reversible fluorescent switching monitored at 630 nm. ( a ) Fluorescence switching of 1 in the Col 1ro phase on the application of −0.7 V (turquoise line), −1.0 V( magenta line), −1.5 V (blue line) and −2.0 V (black line) for 10 s. ( b ) Repetitive switching cycles of 1 in the Col 1ro phase between −1.0 V for 10 s and 0 V for 60 s (delay time between pulses) and ( c ) −4.0 V for 50 ms and 0 V for 60 s delay time between pulses. ( d ) Fluorescence switching of 2 in the SmA phase between −1.0 and +1.0 V for a step duration of 5 s. Full size image This response is observed for reductive voltages even just below the first reduction potential of the thienoviologens up to about −1.5 V ( Fig. 4a ), strongly indicating that the increase of the fluorescence intensity is due to the formation of the radical cation species. The situation clearly changes at −2.0 V ( Fig. 6a ) where the initial rapid increase of the fluorescence reaches a relative maximum and is followed by a quasi-steady-state emission fluorescence level, occurring as long as the voltage is switched on. Notably, when a 0-V is biased into the cell, the fluorescence starts again rapidly to increase up to a maximum and then it decays back to the baseline value after several seconds ( Fig. 6a ). Qualitatively, a molecular mechanistic hypothesis can be advanced for this behaviour: above the second redox potential, the voltage is sufficiently high to cause the reduction of a high fraction of dications to the neutral state that should be a non-emissive species (see below). Thus, the initial increase of the fluorescence due to the radical cation formation is interrupted by the intervention of the neutral species. In the curve tract where the fluorescence assumes a quasi-steady-state level, there is still a fraction of the radical cation species but also of the non-emissive neutral one. When the voltage is set to 0 V, re-oxidation of the neutral species passes through the formation of the radical cation, which causes the fluorescence to increase again. The last part of the curve is essentially the re-oxidation of this species and follows a kinetics similar to that seen at lower voltages. This mechanism is strongly supported by the fact that for the neutral thienoviologen precursor 5,5′-bis(4-pyridyl)-2,2′-bithiophene, no fluorescent emission in the 500–800-nm range is observed (Φ<10 −4 , measured in dichloromethane (DCM) solution). Electrofluorescence switching can be repeated several times by consecutive on/off switching cycles under very different pulse conditions, showing a very efficient electrofluorochromic response of the materials that can be used for fluorescent intensity modulation ( Fig. 6b,c ). Table 2 summarizes the on/off switching times estimated for the pulse conditions of Fig. 6 . It can be seen that the switching times ( τ ) strongly depend on the pulse conditions used. Table 2 reports also the ΔFL defined as the difference between the fluorescence intensity in the on and off states. It is noteworthy that on states with high ΔFL (>65%) can be achieved either with relatively long pulses (a few seconds) at low voltages (−1 V) or with short pulses (ms) at high voltages (−4 V). The on switching time ( τ on ) can be easily chosen to be very short as in the latter case. After a 0-V is biased into the cell ( Fig. 6a–c ) the off state is comparatively reached more slowly ( τ off > τ on ). In such cases, the fluorescent baseline value is spontaneously reached under no driving voltage conditions and the rate-limiting process should be the anion migration essentially for complete re-oxidation of the material to the dication species, as already underlined for the electrochromic response. However, the kinetics of the off state can be very much improved when a complete sweep cycle between negative and positive voltages is applied ( Fig. 6d ). In this case, τ off becomes essentially equal to τ on and is therefore much shorter than the τ off measured in the conditions b being the contrast similar ( Table 2 ). In the alternating electrofluorescence pattern shown in Fig. 6d , each fluorescence increase occurs in the switching on scan (−1 V) on electroreduction of the dication species at the electrode illuminated by the excitation source. In contrast, in the return sweep cycle (switching off at +1 V), the reduced species is re-oxidized to the dication state on the same electrode, leading to a decrease of the fluorescence. This last process is as fast as that leading to electroreduction, which explains the same kinetics of the on and off states. Moreover, when a complete return sweep cycle is performed, device reversibility is much improved, as can be seen by inspection of Fig. 6b–d and by the smaller s.d. of fluorescence contrast and switching times obtained in these conditions ( Table 2 ). Table 2 Switching times of the electrofluorescence. Full size table Considering the fluorescence switching performances of other electrofluorochromic devices under similar step duration and fluorescence contrasts, the switching times reported in Table 2 (row d) are comparable to those reported by Kuo and colleagues ( τ on =4.33 s; τ off =4.22 s) [30] and are even shorter than those estimated from others ( τ on ~8 s; τ off ~7 s) [10] , [31] . These relatively short switching times suggest a fast materials’ reduction due to an efficient electron transport via π–π intermolecular interactions, specifically allowed by the anisotropic nature of the mesophase of the thienoviologens. In summary, here we have presented π-conjugated ILCs exhibiting high fluorescent quantum yields in the bulk state. These materials have unique bulk optical and electrical properties characterizing them as multifunctional nanostructured materials. Indeed, because of their redox electron acceptor moiety, their optical absorption and emission properties can be easily switched by the application of dc electric fields, leading to electrochromism and electrofluorochromism. It is worth noting that, while bulk electrochromism has already been observed in smectic phases, it has never been observed in columnar liquid crystals. Moreover, to the best of our knowledge, bulk electrofluorochromism in liquid crystals has never been reported yet. Interestingly, in the case of compound 2 , the SmA mesophases can be induced by applying an electric field on the isotropic liquid phase; this allows for colour tuning since the emission band of the organized phase is hardly red shifted with respect to that of the Iso state. In conclusion, this study opens the way for developing a new generation of LCs-based electrically modulated optical devices. Sample preparation Compounds 1 and 2 were synthesized as described elsewhere [25] . Bulk electrochemical and optical material properties were investigated in a liquid crystal cell made by sandwitching two ITO glass electrodes. The cell gap was set by means of glass cylinders. Cells were filled by capillary action with the compound in the Iso. Under planar alignment conditions, on cooling from the Iso state the LC molecules spontaneously align parallel to the electrodes surface with columns and smectic layers perpendicular to the electrodes. Electrochemical measurements in solution Cyclic voltammetry of compounds 1 and 2 (1 mM) were acquired in dichloromethane degassed solutions containing 0.1 M tetra- n -butylammonium perchlorate as an electrolyte. Measurements were done at a platinum working electrode in a three-electrode cell, using a platinum auxiliary electrode, an Ag/AgCl reference electrode and a potentiostat configuration from AMEL s.r.l. (Mod. 7050). Scan speed was 30 mV s −1 . Electrochemical and spectroscopic measurements in the bulk Standard cyclic voltammetry was performed with a three-electrode liquid crystal cell (cell gap 40 μm) made of two ITO plates and an Ag wire placed between them, respectively, used as working, counter and reference electrodes ( Fig. 3a ). Electronic spectra were acquired in a two-electrode liquid crystal cell (without the Ag reference) with cell gap of about 7 μm. ITO cells were placed into a Linkam hot stage (LTS350 stage, TP94 System Controller) with internal electrical contacts for simultaneous temperature and dc voltage control. Spectra were recorded with a Jasco V-550 ultraviolet–visible spectrophotometer and dc voltages were supplied by an Amel 2049 model potentiostat. Electrochemical measurements were performed with an Amel Instruments 7050 model potentiostat. Polarizing optical microscopy POM images were acquired with a Leitz Laborlux 12 POL polarizing optical microscope connected to a Lumix Panasonic DMC-FS42 photocamera. Dynamic ionic conductivity measurement Ionic conductivity measurements were performed with a Solartron SI 1260 impedance analyser in the frequency range 10 MHz–0.1 Hz at an applied voltage of 0.3 V. Measurements were performed in the liquid crystalline phase after cooling from the Iso state. Supplementary Figure 3 displays a representative impedance spectrum of 1 at 120 °C where a high frequency relaxation process ( relaxation frequency ~400 Hz) and an incomplete low frequency one can be seen. The first process is attributed to the bulk resistance of the material ( R b ) while the latter is associated with the charge transfer resistance of the interface between sample and electrode [26] , [27] , [28] , [29] . Ionic conductivity ( σ ) was calculated using the equation (1): where K cell is the cell constant given by the ratio between cell gap and electrode area [26] , [27] , [28] , [29] . R b was obtained from the semicircle diameter on the real axis (Z′) ( Supplementary Fig. 3 ) by fitting the experimental spectral points with two resistance-capacitor (RC) circuits in series [26] , [27] , [28] , [29] . Photophysical measurements Spectrofluorimetric grade solvents were used for the photophysical investigations in solution, at room temperature. A Perkin Elmer Lambda 900 spectrophotometer was employed to obtain the absorption spectra. Steady-state emission spectra were recorded on a HORIBA Jobin-Yvon Fluorolog-3 FL3-211 spectrometer equipped with a 450-W xenon arc lamp, double-grating excitation and single-grating emission monochromators (2.1 nm mm −1 dispersion; 1,200 grooves mm −1 ) and a Hamamatsu R928 photomultiplier tube. The ITO sandwich, containing the LC film sample, is placed into the fluorimeter sample holder on a customized temperature-controlled hot stage realized in Teflon by CaLCTec s.r.l. (Rende, Italy), with an uncertainty on the temperature of 1 °C. Measurements were performed in a front-face geometry. Electrofluorochromic measurements were performed by injecting electrons from the ITO surface illuminated by the excitation source to detect the fluorescence response of the first electroreduced layers of the materials. Emission and excitation spectra were corrected for source intensity (lamp and grating) and emission spectral response (detector and grating) by standard correction curves. Time-resolved measurements were performed using the time-correlated single-photon-counting option on the Fluorolog 3. Laser Nanoled at 379 nm, full width half maximum 750 ps, with repetition rate at 1 MHz, was used to excite the sample. Excitation sources were mounted directly on the sample chamber at 90° to a single-grating emission monochromator (2.1 nm mm −1 dispersion; 1,200 grooves mm −1 ) and collected with a TBX-04-D single-photon-counting detector. The photons collected at the detector are correlated by a time-to-amplitude converter to the excitation pulse. Signals were collected using an IBH Data Station Hub photon-counting module, and data analysis was performed using the commercially available DAS6 software (HORIBA Jobin-Yvon IBH). Goodness of fit was assessed by minimizing the reduced χ 2 -function and visual inspection of the weighted residuals. The emission quantum yields of the samples were obtained by means of a Labsphere optical Spectralon integrating sphere (diameter 102 mm), which provides a reflectance >99% over 400–1,500 nm range (>95% within 250–2,500 nm). The sphere accessories are made from Teflon (rod and sample holders) or Spectralon (baffle). The sphere is mounted in the optical path of the spectrofluorimeter using, as excitation source, a 450-W xenon lamp coupled with a double-grating monochromator for selecting wavelengths. Cylindrical tubes containing the solution samples are placed into the sphere, while the ITO sandwich, containing the LC film sample, is placed into the sphere on a customized temperature-controlled hot stage realized in Teflon by CaLCTec s.r.l. (Rende, Italy), with an uncertainty on the temperature of 1 °C. The procedure used to determine the emission quantum yield is based on the de Mello method [32] slightly modified [33] , [34] . The emission quantum yield determination is given by: where A is the value of the absorbance of the sample at the excitation wavelength measured as where L a is the integrated excitation profile when the reference sample is diffusely illuminated by the integrated sphere’s surface; L c is the integrated excitation profile when the sample is diffusely illuminated by the integrated sphere’s surface; E c and E a are the integrated luminescence (corrected for the detector wavelength response) of the sample and the reference sample, respectively, caused by indirect illumination from the sphere. The reference sample is an empty ITO sandwich. The experimental uncertainties were 1 nm for the band maxima of the luminescence spectra and 5% for the emission quantum yield values. How to cite this article: Beneduci, A. et al. Electrofluorochromism in π-conjugated ionic liquid crystals. Nat. Commun. 5:3105 doi: 10.1038/ncomms4105 (2014).